Pharmacological inhibition of Dock5 prevents osteolysis by affecting osteoclast podosome organization while preserving bone formation Osteoporosis is caused by excessive activity of bone-degrading osteoclasts over bone-forming osteoblast. Standard antiosteolytic treatments inhibit bone resorption by inducing osteoclast loss, with the adverse effect of hindering also bone formation. Formation of the osteoclast sealing zone requires Dock5, a guanine nucleotide exchange factor for the small GTPase Rac, and C21, a chemical inhibitor of Dock5, decreases bone resorption by cultured osteoclasts. Here we show that C21 directly inhibits the exchange activity of Dock5 and disrupts osteoclast podosome organization. Remarkably, C21 administration protects mice against bone degradation in models recapitulating major osteolytic diseases: menopause, rheumatoid arthritis and bone metastasis. Furthermore, C21 administration does not affect bone formation and is not toxic. Our results validate the pharmacological inhibition of Dock5 as a novel therapeutic route for fighting osteolytic diseases while preserving bone formation. Excessive osteoclast activity, characteristic of numerous osteolytic diseases, decreases bone strength and increases fracture risk [1] . The most widely used antiosteolytic treatments are nitrogen-containing bisphosphonates, which induce osteoclast apoptosis, and denosumab, a humanized monoclonal antibody to RANKL that inhibits osteoclast differentiation. An important issue with those treatments is that they also strongly affect bone formation [2] . This is suspected to contribute to clinical complications such as atypical subtrochanteric femur fractures and osteonecrosis of the jaw and reduce responsiveness to the bone anabolic factor parathyroid hormone [3] , [4] , [5] . In fact, osteoclasts, even when not resorbing the bone, secrete factors such as afamin, sphingosine-1 phosphate, BMP6 and Wnt10a [6] , [7] , [8] , which stimulate the recruitment and activity of osteoblasts [9] . Novel therapeutic strategies are therefore needed to inhibit osteoclast activity without altering their viability. Osteoclasts adhere on bone by a pososome-based specialized structure: the sealing zone, which delimits the zone of bone resorption [10] . Genetic suppression of genes required for its formation results in higher bone mass in vivo with normal osteoclast differentiation, as we observed in Dock5 −/− mice [11] . Dock5 expression is mainly restricted to osteoclasts and its knockout does not affect mouse survival and breeding while hindering podosome organization into a sealing zone and then bone degradation by cultured osteoclasts [11] , without affecting longitudinal bone growth [12] . We identified C21, a chemical compound blocking Rac activation by Dock5 in cultured cells that inhibits bone degradation by osteoclasts in vitro [11] . The aim of the present study was to use this compound as a model to test whether targeting the osteoclast podosome patterning via the pharmacological inhibition of Dock5 could prevent pathological bone loss while preserving bone formation. Using three mouse models for the most common osteolytic diseases, we show here that systemic administration of the inhibitor of Dock5 efficiently prevents pathological bone loss while preserving bone formation. C21 is a direct inhibitor of Rac activation by Dock5 To establish the molecular basis for the observed inhibition of osteoclastic bone resorption by C21, we first analysed whether C21 was a direct inhibitor of mouse Dock5 catalytic activity. Nucleotide exchange was assayed by fluorescence kinetics using a highly purified Dock5 construct encompassing its previously described DHR2 (DOCK homology region 2) catalytic and dimerization domain [13] and the GTPases Rac1, Rac2, RhoA and Cdc42 ( Supplementary Fig. 1a,b ). Dock5-DHR2 was highly active towards Rac1 ( k cat / K M =7.9±0.33 × 10 4 M −1 s −1 ) and Rac2 ( k cat / K M =9.5±0.35 × 10 4 M −1 s −1 ) ( Fig. 1a and Supplementary Fig. 2a,b ) and had no activity towards RhoA and Cdc42 ( Supplementary Fig. 2a ), indicating that it is strictly specific for the Rac subfamily. C21 inhibits Dock5-DHR2-stimulated nucleotide exchange on Rac1 ( Fig. 1a , red and blue curves) but has no effect on the spontaneous nucleotide exchange rate of the GTPase ( Fig. 1a , green and magenta curves). These biochemical data thus support that C21 is a direct inhibitor of Dock5 function acting through its Rac guanine nucleotide exchange activity. 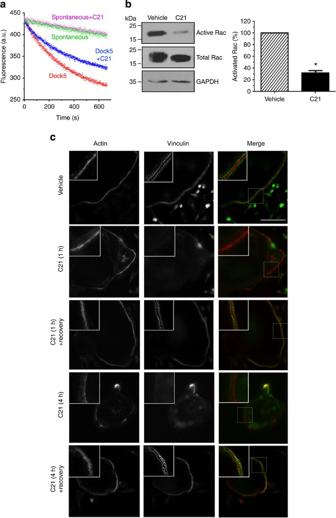Figure 1: Effect of C21 on Rac activation and podosome organization. (a) C21 inhibits activation of Rac1 by DOCK5 but not Rac1 spontaneous GDP/GTP exchangein vitro. Representative fluorescence kinetics curves of Dock5-DHR2-stimulated Rac1 nucleotide exchange in the presence (blue,kobs=29±0.1 10−4s−1) or absence of 50 μM C21 (red,kobs=35±0.4 10−4s−1) and of spontaneous Rac1 nucleotide exchange in the presence (magenta) or absence (green) of 50 μM C21. Experiments were carried out using purified recombinant proteins. a.u., arbitrary unit. All experiments were carried out at least in triplicate. (b) Western blot showing total and active Rac in osteoclasts treated for 1 h with vehicle or 100 μM C21. Bar graph shows mean±s.e.m. per cent of active Rac normalized to total Rac from three independent experiments; *P<0.05, one-tailed Mann–Whitney test. (c) Representative staining actin (red) and vinculin (green) in osteoclasts treated with vehicle or 100 μM C21, for 1–4 h, followed or not by overnight recovery. Scale bar, 50 μM. Insets in merged images show high magnifications of boxes areas. This experiment was performed three times. Figure 1: Effect of C21 on Rac activation and podosome organization. ( a ) C21 inhibits activation of Rac1 by DOCK5 but not Rac1 spontaneous GDP/GTP exchange in vitro . Representative fluorescence kinetics curves of Dock5-DHR2-stimulated Rac1 nucleotide exchange in the presence (blue, k obs =29±0.1 10 −4 s −1 ) or absence of 50 μM C21 (red, k obs =35±0.4 10 −4 s −1 ) and of spontaneous Rac1 nucleotide exchange in the presence (magenta) or absence (green) of 50 μM C21. Experiments were carried out using purified recombinant proteins. a.u., arbitrary unit. All experiments were carried out at least in triplicate. ( b ) Western blot showing total and active Rac in osteoclasts treated for 1 h with vehicle or 100 μM C21. Bar graph shows mean±s.e.m. per cent of active Rac normalized to total Rac from three independent experiments; * P <0.05, one-tailed Mann–Whitney test. ( c ) Representative staining actin (red) and vinculin (green) in osteoclasts treated with vehicle or 100 μM C21, for 1–4 h, followed or not by overnight recovery. Scale bar, 50 μM. Insets in merged images show high magnifications of boxes areas. This experiment was performed three times. Full size image C21 reversibly disrupts podosome organization in osteoclasts We next analysed whether C21 could recapitulate the inhibition of Rac activation and disruption of podosome patterning observed on Dock5 knockdown [11] . Mouse bone marrow-derived osteoclasts were treated with 100 μM C21 and monitored the activation of Rac and the organization of podosomes. After 1 h, the level of active Rac was strongly reduced ( Fig. 1b ) and vinculin showed less pronounced association with actin-labelled podosomes ( Fig. 1c , C21; 1 h). Further incubation for 4 h led to the complete disruption of podosome organization in all osteoclasts ( Fig. 1c , C21; 4 h). Washing out of C21 allowed recovery of normal podosome patterning ( Fig. 1c , recovery). Together, these observations suggest that C21 inhibition of bone degradation by osteoclasts is due to its inhibition of Rac activation by Dock5, which results in impaired podosome organization. C21 is thus a relevant model molecule to test for the effect of pharmacological inhibition of Dock5 on pathological bone loss. For this, we used three mouse models that recapitulate different pathological situations associated with increased osteoclast activation: post-menopause osteoporosis [14] , chronic inflammation [15] and cancer metastasis to the bone [16] . C21 shows no toxic effect in the mouse To assess whether C21 administration could have detrimental effects in the mouse, we initially treated healthy 7-week-old C57Bl/6J mice with vehicle or 25 mg of C21 per kg body weight, 5 days a week, for 4 weeks ( Supplementary Fig. 3a ). As intraperitoneal and intravenous injection routes resulted in similar C21 bioavailability ( Supplementary Fig. 3b ), we used the former in all further experiments. We did not observe any change in body weight ( Supplementary Fig. 3c ), fur ruffling and general activity of C21-treated mice. Moreover, blood analysis showed normal haematocrit ( Supplementary Fig. 3d ), white blood cell counts ( Supplementary Fig. 3e ) and aspartate transaminase activity ( Supplementary Fig. 3f ) and creatinine concentration ( Supplementary Fig. 3g ), suggesting that C21 did not cause allergic reaction or liver and kidney toxicity in mice. Thus, C21 systemic injection has no adverse effects in the mouse. Dock5 inhibition prevents ovariectomy-induced bone loss We first assessed the effect of C21 on post-menopause osteoporosis, which is caused by oestrogen loss [14] and can be reproduced in mice following bilateral ovariectomy (OVX) [17] . We first tested a preventive effect of C21 on bone loss by injecting daily doses of C21 or vehicle to OVX to young adult mice for 4 weeks ( Fig. 2a ). The efficiency of OVX was assessed through the marked reduction in uterus weight ( Supplementary Fig. 4a ) due to uterine atrophy ( Supplementary Fig. 4b,c ). As expected, OVX mice treated with vehicle showed substantial trabecular bone loss with higher osteoclast numbers ( Fig. 2b–d ). In contrast, OVX mice treated with C21 showed a trabecular bone volume not significantly different from SHAM-operated animals ( Fig. 2b ). We did not detect any significant effect of C21 on vertebral trabecular BV/TV of OVX animals ( Supplementary Fig. 4d ). Next, we tested whether C21 was also efficient once a significant bone loss had already occurred in young adult mice. To model a curative OVX situation, the 4-week treatment was initiated after the onset of osteoporosis, that is, starting 2 weeks after OVX ( Fig. 2e ), the efficiency of which was assessed as above ( Supplementary Fig. 4e ). After 2 weeks, OVX animals presented significant femur trabecular bone loss ( Supplementary Fig. 4f ). Treatment was then initiated and after 4 weeks, the BV/TV of OVX mice receiving C21 was significantly higher as compared with vehicle-treated animals and not significantly different from the SHAM-operated controls ( Fig. 2f,g ). C21-treated animals had higher trabecular numbers and reduced trabecular separation as compared with vehicle-treated animals ( Supplementary Fig. 4g–i ). We further analysed the evolution of BV/TV specifically during the 4-week treatment. We found that C21-treated animals preserved 77% of trabecular bone, similar to SHAM-operated animals (85%) and significantly more that vehicle-treated animals (55%) ( Fig. 2h ). The levels of bone resorption marker CTx in C21-treated OVX animals were similar to those in SHAM animals and lower than in vehicle-treated OVX animals, suggesting that C21 treatment inhibited bone resorption ( Fig. 2i ). Together, these results suggest that the inhibition of Dock5 can protect from OVX-induced bone loss. 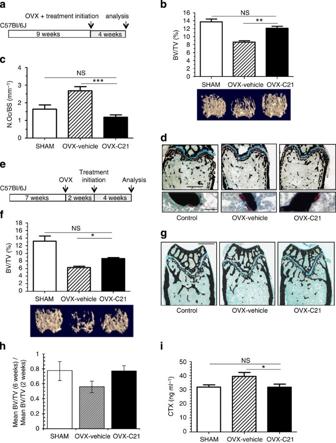Figure 2: C21 protects against ovariectomy-induced bone loss. C57Bl/6J mice were treated with either vehicle or C21, 25 mg kg−1day−1, (a–d) for 4 weeks immediately after ovariectomy (n=13–15 mice per group) or (e–i) between weeks 2 and 6 after ovariectomy (n=10–11 mice per group). (b) Bone volume over total volume (BV/TV) with representative microcomputed tomography images of SHAM-operated (SHAM) mice and ovariectomized (OVX) mice receiving C21 or vehicle. (c) N.Oc/BS, osteoclast number over bone surface determined from the analysis of (d) the region of interest (black dashed lines) of Von Kossa-, alcian blue- and TRAP-stained femur sections; scale bars, 500 μm in top panels and 50 μm in bottom panels. (f) BV/TV with representative microcomputed tomography images SHAM and ovariectomized mice receiving C21 or vehicle and illustrated by (g) Von Kossa and alcian blue stained femur. Scale bar, 500 μM. (h) Bar graph showing ratio between the BT/TV mean at week 6 and the BT/TV mean at week 2, to illustrate bone preservation, with 95% confidence intervals determined with Cauchy’s equation. (i) CTX serum levels at the end of the study. Inb,c,fandi, data are shown as the mean±s.e.m., with NS, not significant; *P<0.05; **P<0.01; ***P<0.001 as determined by Kruskal–Wallis test followed by Dunn’s multiple comparison post-test. Figure 2: C21 protects against ovariectomy-induced bone loss. C57Bl/6J mice were treated with either vehicle or C21, 25 mg kg −1 day −1 , ( a – d ) for 4 weeks immediately after ovariectomy ( n =13–15 mice per group) or ( e – i ) between weeks 2 and 6 after ovariectomy ( n =10–11 mice per group). ( b ) Bone volume over total volume (BV/TV) with representative microcomputed tomography images of SHAM-operated (SHAM) mice and ovariectomized (OVX) mice receiving C21 or vehicle. ( c ) N.Oc/BS, osteoclast number over bone surface determined from the analysis of ( d ) the region of interest (black dashed lines) of Von Kossa-, alcian blue- and TRAP-stained femur sections; scale bars, 500 μm in top panels and 50 μm in bottom panels. ( f ) BV/TV with representative microcomputed tomography images SHAM and ovariectomized mice receiving C21 or vehicle and illustrated by ( g ) Von Kossa and alcian blue stained femur. Scale bar, 500 μM. ( h ) Bar graph showing ratio between the BT/TV mean at week 6 and the BT/TV mean at week 2, to illustrate bone preservation, with 95% confidence intervals determined with Cauchy’s equation. ( i ) CTX serum levels at the end of the study. In b , c , f and i , data are shown as the mean±s.e.m., with NS, not significant; * P <0.05; ** P <0.01; *** P <0.001 as determined by Kruskal–Wallis test followed by Dunn’s multiple comparison post-test. Full size image Dock5 inhibition prevents inflammation-induced bone loss We then evaluated the effect of C21 on bone loss associated with rheumatoid arthritis, a disease characterized by chronic inflammation and synovial hyperplasia in joints that ultimately leads to systemic osteoporosis stimulated by proinflammatory cytokines [15] . It can be modelled by immunization of susceptible DBA/1 mouse strain with type II collagen, the major protein component of articular cartilage [18] ( Fig. 3a ). Both vehicle- and C21-treated mice showed high levels of anti-collagen immunoglobulins ( Fig. 3b ) and developed a rapid inflammation assessed by paw arthritic scoring ( Fig. 3c ), indicating that C21 did not have a direct effect on the inflammatory disease. In contrast, talus BV/TV was significantly higher in arthritic mice treated with C21 as compared with those receiving vehicle and similar to that of naive mice ( Fig. 3d ). In our experimental conditions, C21 had no effect on vertebral trabecular BV/TV ( Supplementary Fig. 4j ). Thus, our results suggest that inhibition of Dock5 can protect mice from bone erosion in the arthritic context through its action on osteoclasts. 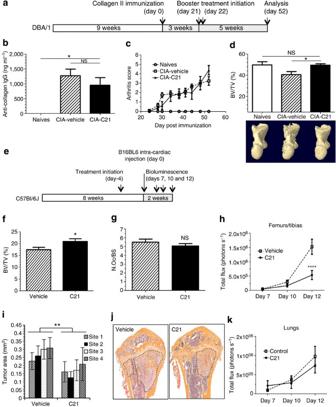Figure 3: C21 protects against arthritis- and metastasis-induced bone loss. Effects of C21 in mouse models of (a–d) bovine collagen-induced arthritis (CIA,n=12–15 mice per group; naivesn=4) and (e–k) osteolytic bone metastasis (n=9–10 mice per group). (a) After bovine collagen injections at days 0 and 21, (b) serum anti-collagen gamma immunoglobulins (IgG) concentration at day 52, (c) evolution of mean clinical arthritic scores and (d) bone volume over total volume (BV/TV) with representative microcomputed tomography images at day 52, in the talus of control mice (naives) and animals treated with vehicle (CIA-vehicle) or C21 (CIA-C21). (e) B16BL6 tumour cells were injected in the left cardiac ventricle of control- (vehicle) or C21- (C21) treated C57Bl/6J mice. (f) Microcomputed tomography assessment of proximal tibia BV/TV. (g) N.Oc/BS, osteoclast number over bone surface. (h,k) B16BL6 cell growth was monitored by photon flux quantification in (h) femurs/tibias and (k) lungs between days 7 and 12. (i) Tumour area in four different matching sections (site 1–4) measured at the end of the study from (j) images of modified haematoxylin- and eosin-stained tibial bone sections (tumours highlighted by dashed lines). Scale bar, 50 μm. Inb–d,f–iandk, graphs show mean±s.e.m. NS, not significant; *P<0.05; **P<0.01; ****P<0.0001 as determined inb,dby Kruskal–Wallis test followed by Dunn’s multiple comparison test, inf,gby two-tailed Mann–Whitney test, iniby pairedt-test and inc,h,kby two-way analysis of variance followed by Bonferroni multiple comparison test. Figure 3: C21 protects against arthritis- and metastasis-induced bone loss. Effects of C21 in mouse models of ( a – d ) bovine collagen-induced arthritis (CIA, n =12–15 mice per group; naives n =4) and ( e – k ) osteolytic bone metastasis ( n =9–10 mice per group). ( a ) After bovine collagen injections at days 0 and 21, ( b ) serum anti-collagen gamma immunoglobulins (IgG) concentration at day 52, ( c ) evolution of mean clinical arthritic scores and ( d ) bone volume over total volume (BV/TV) with representative microcomputed tomography images at day 52, in the talus of control mice (naives) and animals treated with vehicle (CIA-vehicle) or C21 (CIA-C21). ( e ) B16BL6 tumour cells were injected in the left cardiac ventricle of control- (vehicle) or C21- (C21) treated C57Bl/6J mice. ( f ) Microcomputed tomography assessment of proximal tibia BV/TV. ( g ) N.Oc/BS, osteoclast number over bone surface. ( h , k ) B16BL6 cell growth was monitored by photon flux quantification in ( h ) femurs/tibias and ( k ) lungs between days 7 and 12. ( i ) Tumour area in four different matching sections (site 1–4) measured at the end of the study from ( j ) images of modified haematoxylin- and eosin-stained tibial bone sections (tumours highlighted by dashed lines). Scale bar, 50 μm. In b – d , f – i and k , graphs show mean±s.e.m. NS, not significant; * P <0.05; ** P <0.01; **** P <0.0001 as determined in b , d by Kruskal–Wallis test followed by Dunn’s multiple comparison test, in f , g by two-tailed Mann–Whitney test, in i by paired t -test and in c , h , k by two-way analysis of variance followed by Bonferroni multiple comparison test. Full size image Dock5 inhibition prevents metastasis-induced bone loss We then tested the effect of C21 in the context of osteolytic bone metastases where osteoclasts play an adverse role on tumour cell growth. Bone metastases are characterized by the establishment of a vicious cycle where tumour cells activate osteoclasts. In turn, osteoclasts release growth factors by degrading the bone matrix, which increases the proliferation of mestastatic cells in the bone marrow [16] . As the immune system has a versatile role on tumour growth [19] and strongly interplays with the skeletal system [20] , we used a C57Bl/6J syngeneic model system to assay for the effect of C21 on tumour-associated bone loss. We induced osteolytic bone metastases using luciferase-expressing B16BL6 cells derived from B16F10 C57Bl/6J mouse melanoma cells known to have a high tropism for bone [21] , [22] . B16BL6 cells were injected into the arterial system of C57Bl/6J mice via the left cardiac ventricle, and tumour burden was assessed by in vivo bioluminescence imaging at days 7, 10 and 12, following cell inoculation ( Fig. 3e ). Remarkably, mice treated with C21 had higher proximal tibia BV/TV as compared with vehicle controls ( Fig. 3f ) and had similar osteoclast numbers ( Fig. 3g ). Interestingly, these mice also had a significantly lighter tumour burden in the bone ( Fig. 3h–j ). The compound did not affect metastatic cell growth in the lung ( Fig. 3k ), indicating that C21 does not act through an effect on metastatic cell proliferation. These data suggest that the inhibitor of Dock5 acts on bone metastases via the inhibition of bone degradation by osteoclasts, thus breaking the vicious cycle between osteoclasts and metastatic cells in the bone. Dock5 inhibition preserves bone formation Patients exposed to long-term treatment with bisphosphonates have a low bone formation that may in particular increases their susceptibility to atypical femoral fractures [23] . Thus, we finally tested the effect of C21 on bone formation. We first measured bone formation parameters in the context of the above OVX curative model, which reflects the usual treatment initiation after the onset of the disease. We found that C21 treatment did not alter osteoblast numbers ( Fig. 4a ) and activity, as shown by mineral apposition and bone formation rates ( Fig. 4b,c ) and dosage of serum P1NP bone formation marker ( Fig. 4d ). We further compared the effect of C21 with that of the nitrogen-containing bisphosphonate alendronate, a common drug used in the treatment of osteoporosis, by treating healthy mice with vehicle, C21 or alendronate for 4 weeks. In contrast to alendronate, which severely impaired bone formation parameters ( Fig. 4e–i ), C21 did not alter osteoblast numbers ( Fig. 4e ), mineral apposition and bone formation rates ( Fig. 4f–h ) and serum P1NP levels ( Fig. 4i ). It also did not affect osteoclast numbers ( Fig. 4j,k ), BV/TV ( Fig. 4l ), bone mineral density ( Fig. 4m ) and other trabecular bone parameters ( Fig. 4n–p ) as opposed to alendronate. This suggests that inhibiting bone degradation via the inhibition of Dock5 preserves osteoclasts and osteoblasts communication, thus allowing the maintenance of bone formation. 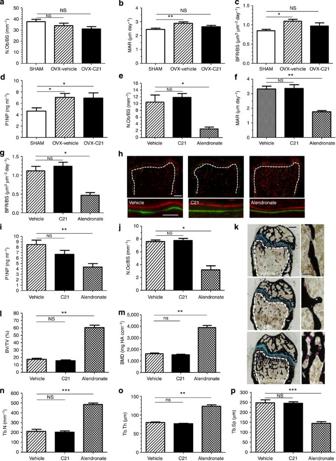Figure 4: C21 does not affect bone formation. Bone formation and histomorphometry analyses of C57Bl/6J mice (a–d) treated with either vehicle or C21, between weeks 2 and 6 after ovariectomy (n=10–11 mice per group), according toFig. 2e, and (e–p) treated with vehicle, C21 or alendronate for 4 weeks (n=5–8 mice per group). In distal femur, (a,e) osteoblast number over bone surface (N.Ob/BS). (b,f) mineral apposition rate (MAR) and (c,g) bone formation rate over bone surface (BFR/BS) determined by quantification of (h) the region of interest (dashed white lines) of calcein (green) and alizarin complexone (red)-labelled sections. Scale bar, 250 μm (top) or 20 μm (bottom). (d,i) P1NP serum concentration. (j) N.Oc/BS, osteoclast number over bone surface from the analysis of (k) the region of interest (white dashed lines) of Von Kossa-, alcian blue- and TRAP-stained femur sections. Scale bar, 300 μm (left panels) and 100 μm (right panels). Microcomputed tomography assessment of (l) BV/TV (m) bone mineral density (BMD), (n) trabecular number (Tb.N), (o) trabecular thickness (Tb.Th) and (p) trabecular spacing (Tb.Sp). All data ina–g,i–jandl–pare shown as the mean±s.e.m. NS, not significant; *P<0.05; **P<0.01; ***P<0.001; determined by Kruskal–Wallis test followed by Dunn’s multiple comparison test. Figure 4: C21 does not affect bone formation. Bone formation and histomorphometry analyses of C57Bl/6J mice ( a – d ) treated with either vehicle or C21, between weeks 2 and 6 after ovariectomy ( n =10–11 mice per group), according to Fig. 2e , and ( e – p ) treated with vehicle, C21 or alendronate for 4 weeks ( n =5–8 mice per group). In distal femur, ( a , e ) osteoblast number over bone surface (N.Ob/BS). ( b , f ) mineral apposition rate (MAR) and ( c , g ) bone formation rate over bone surface (BFR/BS) determined by quantification of ( h ) the region of interest (dashed white lines) of calcein (green) and alizarin complexone (red)-labelled sections. Scale bar, 250 μm (top) or 20 μm (bottom). ( d , i ) P1NP serum concentration. ( j ) N.Oc/BS, osteoclast number over bone surface from the analysis of ( k ) the region of interest (white dashed lines) of Von Kossa-, alcian blue- and TRAP-stained femur sections. Scale bar, 300 μm (left panels) and 100 μm (right panels). Microcomputed tomography assessment of ( l ) BV/TV ( m ) bone mineral density (BMD), ( n ) trabecular number (Tb.N), ( o ) trabecular thickness (Tb.Th) and ( p ) trabecular spacing (Tb.Sp). All data in a – g , i – j and l – p are shown as the mean±s.e.m. NS, not significant; * P <0.05; ** P <0.01; *** P <0.001; determined by Kruskal–Wallis test followed by Dunn’s multiple comparison test. Full size image The prevalence of osteolytic diseases is increasing worldwide, in particular due to general population ageing. The long-term use of current treatments that target the bone-resorbing activity of osteoclasts is associated with more cases of clinical complications due to osteoclast loss, which calls for alternative pharmacological approaches. Here we used a small chemical compound, which can reversibly perturbs podosome organization in osteoclasts through the direct inhibition of Dock5 guanine nucleotide exchange activity. We demonstrate that perturbing the osteoclast bone-resorbing apparatus does not affect bone formation in the mouse and efficiently protects from bone degradation in three osteolytic disease models. We obtained these results through daily systemic administration of a small chemical compound at a relatively small dose. Our findings thus open the route to promising potential therapeutic applications leading to the development of Dock5 chemical inhibitors as novel antiosteolytic treatments that preserve bone formation. Animals Four- to 5-week-old C57Bl/6J and DBA/1 mice were purchased from Harlan (Gannat, France). They were maintained on a 12/12 light/dark cycle, with food and water ad libitum at the CNRS and the IRCM animal facilities in Montpellier, France. All procedures were performed in compliance with the guidelines of the French government and were approved by the Ethic Committee of Languedoc Roussillon (CEEA LR France number 36) for animal experiments under the numbers CEEA-LR-12038 and CEEA-LR-12108. Mice were euthanized by cervical dislocation. C21 C21=N-(3,5-dichlorophenyl)-benzenesulfonamide was synthetized by Roowin (Paris, France) to 99.5% purity ( Supplementary Fig. 5 ). It was dissolved in dimethylsulphoxide for nucleotide exchange assays. For all other experiments, the appropriate amount of C21 was dissolved in 100% ethanol and diluted 1:1 solutol HS15 (Sigma Aldrich, Lyon, France), the resulting mix was further diluted 1:10 in water to obtain a 5% ethanol, 5% solutol C21 solution. OVX-induced osteoporosis C57BL/6J females were fed with soja-free rodent chow (Safe, France) starting 2 weeks before OVX and until sacrifice. Nine-week-old C57Bl/6J females were subjected to either bilateral OVX ( n =27 mice) or sham operation (SHAM, n =15 mice) and treated from the following day with 100 μl intraperitoneal injections of 25 mg C21 per kg body weight ( n =13 OVX-C21 mice) or vehicle ( n =14 OVX-vehicle and 15 SHAM mice), 5 days a week, for 4 weeks. Alternatively, 7-week-old C57Bl/6J females were ovariectomized ( n =32 mice) or sham operated ( n =21 mice) and left untreated for 2 weeks. Eleven mice of each group were killed as baseline control to determine bone loss before treatment initiation. The remaining mice received daily intraperitoneal injections of 25 mg C21 per kg body weight ( n =10 OVX mice) or vehicle ( n =11 OVX and 10 SHAM mice), five times a week, for 4 weeks. After killing, femurs were dissected and cleaned, fixed overnight in 3.7% paraformaldehyde and processed for microcomputed tomography. Uteri were dissected, weighed and embedded in paraffin for histological analysis after haematoxylin/eosin staining to control OVX efficiency. Collagen-induced arthritis model For immunization, bovine type II collagen (MD Biosciences) was dissolved at 3 mg ml −1 in 0.05 M acetic acid for 24 h at 4 °C under rotation and emulsified with the same volume of complete (first injection) or incomplete (second injection) Freund’s adjuvant (Thermo, Saint Léon Rot, France) using micro-emulsifying needles (Cadence inc, Cranstone, RI) and glass syringes (Poulten and Graf GmnH, Wertheim, Germany). Nine-week-old DBA/1 males were immunized twice at days 0 and 21 with a 100 μl intradermal injection of the collagen solution, split between the two sites at the tail base. Treatment with 15 mg C21 per kg body weight ( n =15 mice) or vehicle ( n =15 mice) started day 22 and was administered by 100 μl intraperitoneal injections, 5 days a week, for 30 days. Four naive mice were neither immunized nor treated. Hind paw swelling was measured with a high precision electronic caliper twice a week. Arthritis severity was scored as follows: 0=normal, 1=slight swelling (0.1–0.2 mm) and mild erythema, 2=moderate swelling (0.2–0.4 mm) and erythema, 3=pronounced swelling (0.4–0.6 mm), most fingers are affected, and 4=total ankylosis of the paw and the ankle. At the end of the study, blood was collected to prepare serum for anti-collagen IgG dosage and hind paws were cleaned, fixed overnight in 3.7% paraformaldehyde and processed for microcomputed tomography. Bone metastasis and in vivo bioluminescence imaging Eight-week-old C57BL/6J females ( n =20 mice) received 100 μl intraperitoneal injections of 25 mg C21 per kg body weight ( n =10 mice) or vehicle ( n =10 mice), 5 days a week, between days −4 and 12. At day 0, all mice received a 50 μl intracardiac injection, via the left ventricular chamber, of PBS containing 1.10 5 syngeneic B16BL6 cells stably expressing luciferase (a generous gift from P. Balaguer, INSERM U896, Institut de Recherche en Cancérologie de Montpellier, Montpellier, France). Tumour growth was monitored by in vivo bioluminescence imaging on days 7, 10 and 12 after intraperitoneal injection of 100 mg luciferin per kg body weight (PerkinElmer, Villebon-sur-Yvette, France). Mice were shaved to minimize attenuation of light by pigmented hair and total photon flux (photons s −1 ) was measured from a fixed region of interest (exposure 120 s, binning 16, FOV 24, f/stop 1.2, no filter) using a charge-coupled device (IVIS Lumin, PerkinElmer). Mice were removed from the final analysis if necropsy demonstrated a large mediastinal tumour indicative of tumour cell injection into the chest cavity. After mouse killing at day 12, tibias were collected, cleaned, fixed overnight in 3.7% paraformaldehyde, processed for microcomputed tomography and then embedded in paraffin for histological analysis after modified haematoxylin–eosin staining. Tumour area in proximal tibias was measured on four different sections distant from 60 μm and matching between the bones, using Bioquant Osteo II version 12.1.6 (Bioquant Image Analysis, Nashville, TN, USA), with the region of interest defined as 1.7 mm long starting 250 μm from the proximal tibia growth plate. Healthy mice treatment Seven-week-old C57Bl/6J males and females (50:50) received intraperitoneal injections of C21 (25 mg kg −1 per day, 5 days a week), vehicle or alendronate sodium trihydrate (Sigma, 100 μg kg −1 per day, twice a week [24] ), for 4 weeks ( n =10 mice per group). Microcomputed tomography Microcomputed tomography experiments were performed using a Bruker-Skyscan 1076 (Kontich, Belgium) in vivo X-ray microtomograph at Montpellier RIO Imaging platform and LabEx CeMEB facility. In brief, femurs were scanned in 200-μl tubes filled with 70% ethanol at 50 kV and 200 μA with no filter, 0.4 rotation step, frame averaging of 2, ¼ partial width and 9.04 μm pixel size. Hind paws were wrapped in paper towel and immersed in 70% ethanol in 5 ml plastic tubes. They were scanned at 50 kV and 200 μA with a 0.5 mm aluminium filter, a rotation step of 0.3, frame averaging of 2, ¼ partial width and 9.04 μm pixel size. Projection images were reconstructed using Nrecon software (Bruker-Skyscan) and further analyses and three-dimensional visualization were performed using CTan and CTvol softwares (Bruker-Skyscan). The regions of interest were defined in the trabecular zone (avoiding the cortical bone) from 0.5 to 1.9 mm below the femur distal growth plate and from 0.25 to 2.05 mm below the tibia proximal growth plate. Whole talus bones were analysed. Bone formation and histomorphometry Healthy and OVX mice received intraperitoneal injections of 10 mg kg −1 calcein in sodium carbonate 2% and 20 mg kg −1 alizarin complexone, 8 and 2 days before killing, respectively. Femurs were fixed in 3.7% paraformaldehyde and embedded in methyl methacrylate plastic after serial dehydration with a graded ethanol series to xylene. Five-μm sections were directly imaged using a Nanozoomer run by NDPI software (Hamamatsu). Bone histomorphometry was performed with Bioquant Osteo II version 12.1.6 (Bioquant Image Analysis, Nashville, TN). The region of interest was defined as 1.2 mm long starting 100 μm from the distal femur growth plate. We assessed mineral apposition rate and bone formation rate by calcein and alizarin complexone double staining, osteoblast number by Goldner’s trichrome staining and osteoclast number by TRAP/Von Kossa/alcian blue staining. For bone metastasis experiment, tibias were embedded in paraffin, sectioned, stained with TRAP/haematoxylin–eosin staining and analysed for osteoclast numbers in the region of interest defined as 1.7 mm long starting 250 μm from the proximal tibia growth plate. Blood collection, serum preparation and analyses Anesthetized mouse blood samples were collected by retro-orbital puncture. Haematocrit was determined by measuring packed red blood cell percentage in the blood after centrifugation in micro-haematocrit tubes with sodium heparin (Brand, Radebeul, Germany). For white blood cell counts, blood smears were stained with May–Grünwald Giemsa solution (Merck, Fontenay sous Bois, France). Alternatively, blood was allowed to clot at room temperature for 10 min, centrifuged at 1,500 g for 10 min and serum was stored at −20 °C until analysis. Serum aspartate transaminase activity (Enzychrom Aspartate Transaminase Assay kit, BioAssay Systems, Haymard, CA), creatinine (Quantichrom creatinine assay kit, BioAssay Systems), total anti-type II collagen IgG (Mouse IgG anti-bovine collagen type 2 ELISA, MD Bioproducts, Saint Paul, MN) and P1NP (Rat/mouse P1NP EIA, IDS) quantifications were performed following manufacturer instructions. For C21 bioavailability, 8-week-old C57BL/6J male mice received 25 mg C21 per kg body weight either by intraperitoneal or intravenous route ( n =9 mice for each group). Serum samples collected at different time points (1, 5, 15, 30, 45min and 1, 2, 3, 5 h after injection) were stored at −20 °C before mass spectrometry quantification at the mass spectrometry platform from the Institut des Biomolécules Max Mousseron, Montpellier, France. All experiments were carried out on a Waters Acquity chromatographic system (Waters, Milford, MA) and a ThermoFinnigan Ultra-Quantum triplequadrupole mass spectrometer equipped with an electrospray ionization source (ThermoElectron Corporation, Madison, WI). Chromatographic separation was performed on an Eclipse plus C18 column 50 × 2.1 mm, 1.7 μm (Agilent, Massy, France). The column was thermostated at 25 °C. The autosampler tray was maintained at 5 °C. The analytical separation was achieved with a binary elution gradient program. The two eluents were: (A) water and (B) acetonitrile. The mobile phase was delivered at a flow rate of 1 ml min −1 using the following stepwise gradient elution program: from 0 to 100% of B in 5 min. The injection volume was 10 μl. The Ultra-Quantum mass spectrometer operated in negative electrospray ionization and multiple reaction monitoring modes. The instrument was optimized for the compound C21 by infusing at 10 μl min −1 a 10-mg ml −1 solution of analyte diluted in the 50/50 eluents A and B mix. Argon was used as collision gas at 1.5 m Torr. Spray voltage and capillary temperature were set at 3,000 V and 350 °C, respectively. The pressures for the nitrogen sheath gas, auxiliary gas and sweep gas were maintained at 50, 10 and 2 units (units refer to an arbitrary value set by the X-calibur software). The analyte-specific MS parameters and multiple reaction monitoring transitions were as below: Osteoclast differentiation Bone marrow macrophages were isolated from long bones of 6–8-week-old female or male C57Bl/6J mice, as previously described [25] . Non-adherent bone marrow cells were cultured in αMEM containing 10% heat-inactivated foetal calf serum (Life Technologies, Saint Aubin, France) and 2 mM glutamine, supplemented with 30 ng ml −1 macrophage colony-stimulating factor (M-CSF; Peprotech, Neuilly sur Seine, France) for 48 h and used as bone marrow-derived macrophages. For osteoclast differentiation, bone marrow-derived macrophages were cultured in the presence of 100 ng ml −1 RANKL (Peprotech) and 30 ng ml −1 M-CSF, at the density of 6 × 10 4 cells per well (12-well plate) or 1.5 × 10 5 cells per well (six-well plate). Media was changed and cytokines were replenished every 2 days, and cultured for 4–5 days with 30 ng ml −1 M-CSF and 100 ng ml −1 RANKL (Peprotech) to obtain osteoclasts. Active Rac quantification Osteoclasts were differentiated in six-well plates and treated with 100 μM C21 or vehicle for 1 h. Rac was pulled down from differentiated osteoclast cell extracts using GST-fused PAK1 CRIB domain, as described previously [26] . Cells were lysed in 25 mM HEPES (pH 7.5), 1% Igepal, 5% glycerol, 100 mM NaCl, 10 mM MgCl 2 , 5 mM NaF, 1 mM Na3VO4 and Protease Inhibitor Cocktail (Sigma Aldrich, Saint-Quentin-Fallavier, France). Cleared lysate was incubated with 25 μg of GST-Pak CRIB bound to glutathione-coupled Sepharose beads (Tebu Bio, Le Perray-en-Yvelines, France) for 45 min at 4 °C. Beads were washed three times in lysis buffer before addition of Laemmli sample buffer. Rac was revealed by western blot using ECL western reagent (PerkinElmer, Villebon-sur-Yvette, France) with a monoclonal anti-antibody used 1:10,000 (Millipore, Saint-Quentin en Yvelines, France) followed by a secondary antibody to mouse coupled to horseradish peroxidase used 1:10,000 (GE Healthcare Life Science, Vélizy Villacoublay, France) ( Supplementary Fig. 6 ). Quantification of activation was performed by densitometric analysis using ImageJ software. The relative amount of active Rac was determined relative to the total amount of the protein in whole-cell lysates. Immunofluorescence staining Osteoclasts were differentiated on glass coverslips in 24-well plates and treated with 100 μM C21 or vehicle for 1, 2 or 4 h, followed or not by overnight recovery. Cells were fixed with 3.7% paraformaldehyde for 15 min, permeabilized with 0.1% Triton X-100 in PBS for 1 min and stained for actin and vinculin using rhodamine-labelled phalloidin and anti-vinculin monoclonal antibody used 1:100 (Sigma Aldrich, Lyon, France) revealed with Alexa Fluor 488-conjugated anti-mouse secondary antibody used 1:1,000 (Life Technologies, Saint Aubin, France). Preparations were mounted in Mowiol 40–88 (Sigma Aldrich) and imaged with a Zeiss Axioimager Z2 microscope with Coolsnap HQ2 camera for fluorescence using a Zeiss 40_PLAN-NEOFLUAR 1.3 oil DIC (Zeiss, Inc., Thornwood, NY, USA). Images were acquired with MetaMorph 7.6.6 software (Molecular Devices, Sunnyvale, CA). Nucleotide exchange assays The DHR2 domain of mouse Dock5 (residues 1212-1642, Dock5-DHR2, as defined for Dock2 in ref. 13 ) was expressed in Escherichia coli as a 6 × His-MBP fusion with a TEV protease cleavage site. The tag was cleaved and the protein was purified to homogeneity ( Supplementary Fig. 1a ). Dimerization of Dock5-DHR2 was assessed by size-exclusion chromatography coupled to multi-angle light scattering analysis ( Supplementary Fig. 1b ). Full-length human Rac1, Rac2, RhoA and Cdc42 carrying a 6-histidine tag fused to their C-terminus were expressed in E. coli and purified to homogeneity ( Supplementary Fig. 1a ). Small GTPases were loaded with N -methylanthraniloyl-GDP (mant-GDP, JenaBiosciences, Jena Germany) before nucleotide exchange kinetics experiments. Nucleotide exchange kinetics were monitored by fluorescence of the mant fluorophore ( λ exc =360 nm, λ em =440 nm) using a Cary Eclipse fluorimeter (Varian, Toulouse, France) at 30 °C under stirring. All kinetics assays were carried out in a buffer containing 50 mM Tris at pH 8, 300 mM NaCl, 2 mM MgCl 2 , 1 mM DTT, 0.1% dimethylsulphoxide and were started by addition of 100 μM GTP. Nucleotide exchange kinetics were carried out at a concentration of small GTPases of 1 μM, either without Dock5-DHR2 for spontaneous exchange, in the presence of 50 nM Dock5-DHR2 for single k obs (s −1 ) determination, or using a range of Dock5-DHR2 concentrations for k cat / K M (M −1 s −1 ) determination. The k obs and k cat / K M were determined as described [27] from single-exponential fit of the fluorescence change. k cat / K M (M −1 s −1 ) were obtained following a Michaelis–Menten formalism from: k obs =( k cat / K M )[Dock5-DHR2]+ k spont where k spont is the spontaneous nucleotide exchange rate constant. All experiments were carried out at least in triplicate. Statistical analysis We assessed statistical significance with the non-parametric Mann–Whitney test or using the Kruskall–Wallis test followed by Dunn’s post-test, in case of more than two samples. For comparisons including time courses, we used two-way analysis of variance. Paired t -test was used to determine whether there is a significant difference between the tumour areas measured on four different sections of the same tibia. All analyses were performed using GraphPad Prism (GraphPad Software, Inc., La Jolla, CA). P values <0.05 were considered statistically significant. All data are presented as the mean±s.e.m.. Cauchy’s equation was used to determine the confidence intervals of a quotient. How to cite this article: Vives, V. et al . Pharmacological inhibition of Dock5 prevents osteolysis by affecting osteoclast podosome organization while preserving bone formation. Nat. Commun. 6:6218 doi: 10.1038/ncomms7218 (2015).